Second-generation environmental sequencing unmasks marine metazoan biodiversity Biodiversity is of crucial importance for ecosystem functioning, sustainability and resilience, but the magnitude and organization of marine diversity at a range of spatial and taxonomic scales are undefined. In this paper, we use second-generation sequencing to unmask putatively diverse marine metazoan biodiversity in a Scottish temperate benthic ecosystem. We show that remarkable differences in diversity occurred at microgeographical scales and refute currently accepted ecological and taxonomic paradigms of meiofaunal identity, rank abundance and concomitant understanding of trophic dynamics. Richness estimates from the current benchmarked Operational Clustering of Taxonomic Units from Parallel UltraSequencing analyses are broadly aligned with those derived from morphological assessments. However, the slope of taxon rarefaction curves for many phyla remains incomplete, suggesting that the true alpha diversity is likely to exceed current perceptions. The approaches provide a rapid, objective and cost-effective taxonomic framework for exploring links between ecosystem structure and function of all hitherto intractable, but ecologically important, communities. Biodiversity is the product of millions of years of evolution and forms the basis of the earth's life support system, but the magnitude and relative diversity of global species richness remain unknown. On earth, there may be over 100 million species [1] but fewer than two million have been formally described [2] . There is also a pronounced bias towards the study of larger organisms, leaving the most speciose communities that are dominated by microscopic organisms understudied. To study diverse environments dominated by small taxa, second-generation sequencing has been used for the quantification of bacteria, archaea [3] , [4] and viruses [5] , [6] , but large knowledge gaps still exist regarding the organization of diversity within several eukaryotic kingdoms, including the Metazoa [7] . The Kingdom Metazoa, also known as Animalia, consists of multicellular heterotrophic organisms ranging from Porifera to Chordata. Contemporary phylogenetic studies routinely recover a monophyletic Bilateria—Triploblasta clade (including deep-branching Ecdysozoa, Lophotrochozoa and Deuterostomia) [8] , [9] , but no consensus view exists of the precise relationships between Bilateria, and the basal groups of Porifera, Ctenophora, Placozoa, Cnidaria and Coelenterata [8] , [9] . Marine benthic metazoan communities display some of the highest α-diversity on the planet and occupy one of the largest ecosystems on earth, where only 1% of species are estimated to be known [10] . Benthic meiofauna (small metazoans between 45 and 500 μm in size) comprises members encompassing 60% of animal phyla and represents a major part of marine biodiversity [10] . Dominated by nematodes and characterized by high abundances (up to 10 8 individuals per 1 m 2 ) and diversity [11] , meiofaunal assemblages perform essential roles in marine ecosystem processes, namely, nutrient cycling, secondary production, sediment transport and mineralization [12] . In this paper, we apply a metagenetic approach (that is, the large-scale analysis of taxon richness through the analysis of homologous genes [7] ) using second-generation sequencing of the 18S nuclear small subunit (nSSU) ribosomal RNA (rRNA) gene to assess simultaneously the relative levels of richness and patterns of diversity of multiple metazoan phyla across an ecological gradient in a temperate benthic ecosystem. The heterogeneous levels of accumulating taxon richness derived from the benchmarked analyses were broadly congruent with those derived from intensive morphological assessments, but MEGABLAST annotation revealed a previously unidentified phylogenetic breadth of microbial metazoan life. Moreover, the finding that the largely predacious turbellarian Platyhelminthes represent a substantial proportion of benthic diversity quantifies their hitherto unrecognized ecological importance in benthic food chains. Annotated metagenetic analyses enable the objective assessment of microbial biodiversity throughout all ecosystems, facilitating understanding of linkages between microbial biodiversity and ecosystem processes. Taxon richness estimates nSSU rRNA amplicons were generated from eight benthic samples from the low-tide zone of an estuarine beach near Prestwick on the West coast of Scotland, and from one sample from a beach in Littlehampton in the South of England. 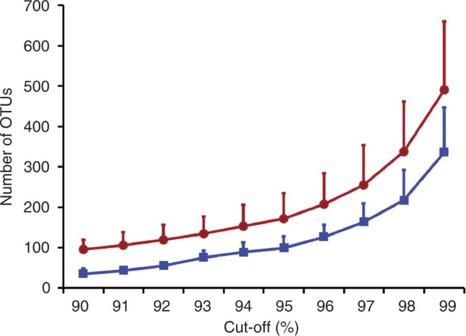Figure 1: Lineage-through-time plots for OCTUPUS and ESPRIT. Mean number of OTUs plotted against each percentage identity cut-off (90–99% similarity) generated using 5,000 subsampled sequences (>199 bases in length) from three independent sample sites (Prestwick 2, 7 and Littlehampton 1) using OCTUPUS (blue squares) and ESPRIT's HCluster13(red circles) OTU clustering. Values are given as average+s.d. (n=9). The amplicons were processed for sequencing on a Roche 454 FLX platform generating a total of 353,896 sequences that were quality filtered to 305,702 for downstream analysis ( Table 1 ). When performing metagenetic assessments of taxon richness, it is important to cluster taxonomic units in a biologically meaningful manner, as even slight differences in similarity cut-offs and using different algorithms can result in significantly different estimates of richness. The taxon clustering comparisons between ESPRIT [13] and OCTUPUS (the Operational Clustering of Taxonomic Units from Parallel UltraSequencing, supplementary software available at http://octupus.sourceforge.net/ ) ( Fig. 1 ) on the subsampled beach pyrosequencing data show that ESPRIT overestimates Operational Taxonomic Units (OTUs) richness compared with OCTUPUS (between 1.1x–4.4x, over the 90–99% cut-off range). Phylogenetic [14] and barcoding [15] studies based on the analysis of chain-termination nSSU gene sequences suggest that intraspecific divergence at least in nematode species is low (1–2%). However, the true level of intragenomic and intraspecific variation among rRNA gene repeats is largely unknown, and genome-wide analyses reveal a dominant set of conserved sequences accompanied by rare variant sequences [16] . Our benchmarking exercise, performed against a reference control data set comprising 41 species [17] , revealed that the 96% similarity OCTUPUS clustering algorithm with accompanying chimera screening estimated taxon richness that was most closely aligned with species richness. At 96% similarity, OCTUPUS resulted in 37 operational clustered taxonomic units (OCTUs), whereas at 97%, OCTUPUS resulted in 51 OCTUs from the control metagenetic analysis [17] . Thus, although we may be underestimating richness by at least 10%, we have opted for a more conservative approach of setting a 96% identity OCTU cut-off for all subsequent numerical comparisons. At this cut-off, an OCTU is likely to (at worst) correspond to a group of related species. Following the 96% similarity OCTUPUS clustering strategy, the total number of putatively non-chimeric tag reads and OCTUs was 217,221 and 428, respectively. Before chimera screening, 1013 OCTUs were clustered from the initial quality-screened 305,702 reads. Table 1 Total number of pyrosequencing sequences after quality control and chimera screening. Full size table Figure 1: Lineage-through-time plots for OCTUPUS and ESPRIT. Mean number of OTUs plotted against each percentage identity cut-off (90–99% similarity) generated using 5,000 subsampled sequences (>199 bases in length) from three independent sample sites (Prestwick 2, 7 and Littlehampton 1) using OCTUPUS (blue squares) and ESPRIT's HCluster [13] (red circles) OTU clustering. Values are given as average+s.d. ( n =9). Full size image Community richness is closely linked to the environment The peak of standardized OCTU richness for all phyla was within samples 6, 7 and 8 from Prestwick, and cluster analyses indicated clear and fine-scale hierarchical distinctions in OCTU composition within and between the two sites, with clear divergence of samples from Littlehampton ( Fig. 2 ). OCTU richness and sediment grain size were clearly correlated (Spearman's correlation coefficient, n =9, ρ =−0.82, P =0.0108). 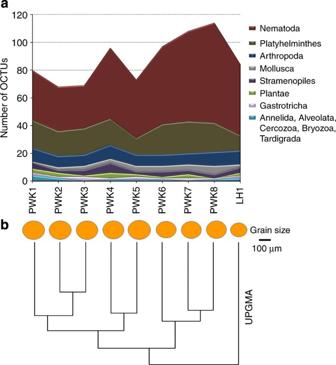Figure 2: Taxon richness and community similarity in relation to ecology and space. (a) Number of different OCTUs per sample for each phylum after data standardization derived from the Prestwick (eight sampling sites) and Littlehampton (one sampling site) marine littoral benthos; (b) grain size represents the relative 50% cumulative median grain size (μm) per site, and cluster analyses (UPGMA) using Sorensen's Coefficient represent the number of shared OCTUs between the nine independent samples. The positive relationship between grain size and sample richness is highly significant (Spearman's correlation coefficient,n=9,ρ=−0.83,P=0.0108). Figure 2: Taxon richness and community similarity in relation to ecology and space. ( a ) Number of different OCTUs per sample for each phylum after data standardization derived from the Prestwick (eight sampling sites) and Littlehampton (one sampling site) marine littoral benthos; ( b ) grain size represents the relative 50% cumulative median grain size (μm) per site, and cluster analyses (UPGMA) using Sorensen's Coefficient represent the number of shared OCTUs between the nine independent samples. The positive relationship between grain size and sample richness is highly significant (Spearman's correlation coefficient, n =9, ρ =−0.83, P =0.0108). Full size image Dominance of the Nematoda and rise of the Platyhelminthes Plotting phylum richness rank for all nine independent samples ( Fig. 3 ) shows that Nematoda are the most OCTU-rich in all nine samples, with Platyhelminthes and Arthropoda ranking second and third in all, respectively. 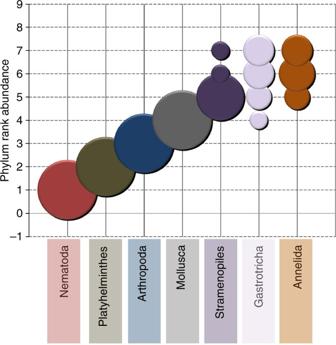Figure 3: Phylum rank abundance plot. Community assemblage OCTU richness rank order for the main phyla recovered from the Prestwick and Littlehampton samples (after data standardization). The frequency of ranking (out of the nine samples) is represented by the diameter of the symbol at each rank. Single symbols per phylum represent a constant ranking, whereas multiple symbols highlight variance in phylum rank order throughout the samples. Figure 3: Phylum rank abundance plot. Community assemblage OCTU richness rank order for the main phyla recovered from the Prestwick and Littlehampton samples (after data standardization). The frequency of ranking (out of the nine samples) is represented by the diameter of the symbol at each rank. Single symbols per phylum represent a constant ranking, whereas multiple symbols highlight variance in phylum rank order throughout the samples. Full size image Annotated metagenetic analyses can yield robust relative richness estimates and here it was possible to assign 374 OCTUs to phylum ( Fig. 4a ). The PCR primers used are not fully specific to Metazoa, and thus we also sequenced nSSU genes from protist taxa from the Alveolata (2 distinct OCTUs), Cercozoa (3 OCTUs) and Stramenopiles (15 OCTUs). Of the metazoan OCTUs, 182 were from Nematoda, at least three times more than from any other individual meiofaunal taxon ( Fig. 4a ). Platyhelminthes (61 OCTUs) was the second richest phylum, followed by Arthropoda (29 OCTUs including Copepoda, Ostracoda and Malacostraca), Mollusca (22 OCTUs), Gastrotricha (7 OCTUs), Annelida (6 OCTUs) and five less-rich phyla (for example, Bryozoa, Echinodermata, Cercozoa, Rotifera and Alveolata with between 1 and 3 OCTUs each). 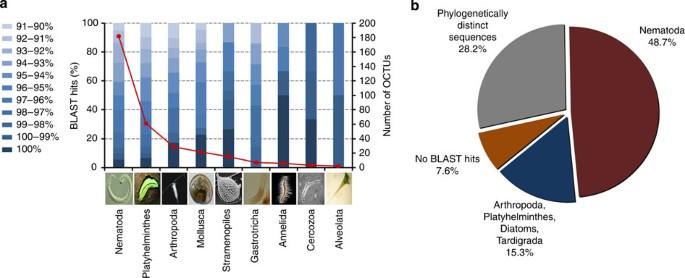Figure 4: Percentage identity to known sequences and number of OCTUs found for the main phyla. (a) Number of different OCTUs for the main phyla recovered from the Prestwick and Littlehampton meiofaunal samples and their different levels of identity to nSSU in the GenBank/EMBL/DDBJ nucleotide database. (b) Putative taxonomic classification of 39 OCTUs that had less than 90% sequence identity to nSSU in GenBank/EMBL/DDBJ. We acknowledge and thank Richard Ling (Platyhelminthes), Frederico Batista (Mollusca), David Mann (Stramenopile), Greg Rouse (Annelida), Charisa Wernick/MicroscopeWorld (Alveolata), Tim Ferrero (Nematoda), Kim Taylor/Warren Photographic (Arthropoda), Graham Matthews (Gastrotricha) and David Bass (Cercozoa), who gave permission to use the images inFigure 4a. Figure 4: Percentage identity to known sequences and number of OCTUs found for the main phyla. ( a ) Number of different OCTUs for the main phyla recovered from the Prestwick and Littlehampton meiofaunal samples and their different levels of identity to nSSU in the GenBank/EMBL/DDBJ nucleotide database. ( b ) Putative taxonomic classification of 39 OCTUs that had less than 90% sequence identity to nSSU in GenBank/EMBL/DDBJ. We acknowledge and thank Richard Ling (Platyhelminthes), Frederico Batista (Mollusca), David Mann (Stramenopile), Greg Rouse (Annelida), Charisa Wernick/MicroscopeWorld (Alveolata), Tim Ferrero (Nematoda), Kim Taylor/Warren Photographic (Arthropoda), Graham Matthews (Gastrotricha) and David Bass (Cercozoa), who gave permission to use the images in Figure 4a . Full size image Metagenetics reveals phylogenetically distinct taxa According to the comparisons of the OCTU sequences with the NCBI database, the majority (95%) of Nematoda OCTUs have never been sequenced before ( Fig. 4a , Table 2 ). Similarly, only 6.5% of Platyhelminthes and 17.2% of Arthropoda OCTUs had 100% identity to previously sequenced specimens. The Annelida, Mollusca and Stramenopiles, however, had 50, 23 and 26.6%, respectively, of their OCTUs, with a 100% identity to previously sequenced taxa. None of the Gastrotricha OCTUs were identical to previously sequenced taxa. Overall, 54 OCTUs (representing 7,247 individual sequences) had identities below 90% to any reference nSSU sequence (OCTUs<90% identity), and may represent previously unsampled diversity. Given the nature of the adopted clustering algorithm, the OCTUs with <90% identity do not show any pattern of variation that would be expected of a chimeric assemblage of the already defined 428 OCTUs. Fifteen of the OCTUs with <90% identity (300 sequences) were robustly placed within identified phyla (mainly Nematoda). A further 36 were either sisters to the sequences from known phyla, or represented deep, likely misplaced branches ( Fig. 4b ). Surprisingly, 11 OCTUs with <90% identity, comprising 107 sequences in total distributed across the sampling area, were not affiliated to any phyla. The similarity of the latter sequences ranged between 83 and 89% to known nSSU genes, suggesting that they may represent unknown, distinct lineages. Furthermore, three OCTUs resulted in no MEGABLAST hit, but two of these exhibited signatures of relaxed selection, indicating that they may represent translocated 'orphan' nSSU genes that are no longer constrained by function. Resampling to generate longer sequences beyond the 200 base pairs presented here will be required to confirm or refute the biological reality of these phylogenetically distinct sequences. Table 2 OCTUs with 100% identity to nSSU sequences in the GenBank/EMBL/DDBJ database. Full size table Metazoan richness curves do not approach saturation Along the Prestwick transect, the slope of OCTU rarefaction curves at 96% cut-off for the Nematoda, Platyhelminthes, Arthropoda, Mollusca, Stramenopiles and Annelida phyla did not reach an asymptote ( Fig. 5 ). However, 217,221 samples and 374 OCTU-defined taxa fail to achieve saturation, even for low abundance phyla in which rareaction curves tend to converge [18] . 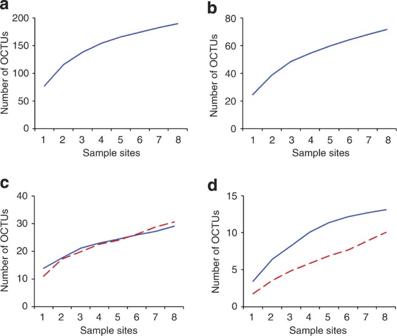Figure 5: Rarefaction curves of the abundance-based coverage estimation (ACE) diversity estimator. Plots are shown for (a) Nematoda, (b) Platyhelminthes, (c) Arthropoda (blue) and Mollusca (red dashed), (d) Stramenopiles (blue) and Annelida (dashed red) at 96% identity OCTU cut-off for the Prestwick meiobenthic samples 1–8. Curves were estimated from 100 randomizations, without replacement, using EstimateS, version 8.2.0. Figure 5: Rarefaction curves of the abundance-based coverage estimation (ACE) diversity estimator. Plots are shown for ( a ) Nematoda, ( b ) Platyhelminthes, ( c ) Arthropoda (blue) and Mollusca (red dashed), ( d ) Stramenopiles (blue) and Annelida (dashed red) at 96% identity OCTU cut-off for the Prestwick meiobenthic samples 1–8. Curves were estimated from 100 randomizations, without replacement, using EstimateS, version 8.2.0. Full size image Both ESPRIT [13] and OCTUPUS can be used to cluster OTUs from the size of the environmental metagenetic data set presented here, without the need of a computing cluster. Nevertheless, ESPRIT may overestimate OTU richness, presumably because it counts both substitutional and independent insertion/deletion (indel) events in OTU clustering. One of the most widely publicized artefacts of 454 Roche pyrosequencing is its inherent inaccuracy in calling homopolymer runs, including extensions (insertions), incomplete extensions (deletions) and carry forward errors (insertions and substitutions) [19] , [20] , [21] . Therefore, clustering algorithms that use indel data informatively, especially as independent events at homologous base positions [22] , are likely to be susceptible to higher OTU estimates. Analyses herein, and those of Sun et al . [13] , suggest that OCTUPUS generates a conservative number of OTUs compared with both ESPRIT and combinations of MUSCLE [23] and DOTUR [24] . Nevertheless, it is imperative, when possible, to benchmark the analytical framework against real or simulated data, in order to estimate taxon richness as realistically as possible [21] . The patterns of taxon richness along the Prestwick transect exhibited remarkable differences even at a microgeographical scale. Although numerous environmental factors influence meiobenthic distribution and assemblage, grain size, examined here, is known to be the predominant driver of meiofaunal community structure and diversity [12] . Nevertheless, the fine-scale community structuring also indicates that there are likely to be a host of additional biotic (for example, prokaryote communities and organic matter) and abiotic (sediment grain shape, surface composition) microgeographical factors responsible for community structuring within the benthos [12] . Nematodes account for approximately 80% of all individual animals on earth, but quantifying the levels of relative richness between major Metazoan phyla has not been practical hitherto, because of the taxonomic magnitude of the challenge. Remarkably, along only an 800 m transect, we detected 182 Nematoda OCTUs, compared with 450 species of Nematode that have been described from around the entire British Isles [25] . From a geographical perspective, these data represent the discovery of 40% of the previously known phylum richness from a transect that represents 0.004% of the length of the British coastline ( ∼ 17,820 km, Ordnance Survey). Molecular definition of substantial meiofaunal taxon richness at microgeographical scales is in alignment with intensive morphological studies [35] , yet recent metagenetic studies from the microbial biosphere have suggested that taxon richness may be orders of magnitude more than previously expected [3] , [4] , [5] , [6] . Reeder and Knight [26] , Quince et al . [27] and Huse et al . [28] have recently provided alternative interpretations, based on pyrosequencing error, DNA recombination and clustering approaches, for earlier studies reporting extensive richness and rare biospheres derived from Roche 454 pyrosequencing. The data here have been quality/size filtered; only substitutional variance has contributed to taxon identification and a particularly aggressive chimera screen has been applied to featured OCTUs. In combination with the benchmarking exercise performed against known taxa, it is therefore highly unlikely that the delineated taxa are based on sequencing error, and taxon estimates are likely to underestimate richness by at least 10%. Although global nematode diversity estimates range from 1 to 100 million species, only 24,000 species have been described [29] , with ∼ 2,000 marine species catalogued in Europe [30] . Such relative paucity of taxonomic knowledge of nematode biodiversity is a product of their numerical dominance, the number of taxa and the high level of cryptic species: this taxon is thus a prime candidate for taxonomic exploration using metagenetic analyses. Why are Nematoda so dominant, in both abundance and diversity, in meiofaunal communities? Benthic nematodes are small in size and possess rapid generation times, and these attributes may have facilitated rapid adaptation to local conditions and habitats, especially in interstitial niches. The taxonomic richness of nematodes is, in addition, likely promoted by ancient ancestry [31] and the absence of a dispersal phase, promoting speciation across structurally and spatially heterogeneous environments during glacial and interglacial periods. Nematodes also have cryptobiotic adaptations, including resting eggs and highly resistant larvae [32] , and they are considered to be especially resistant to environmental challenges, being among the last taxa to disappear in an environmental catastrophe [33] . As no other meiofaunal phylum shares all such characteristics simultaneously, nematodes may have had the time and potential to diversify, endowing them with collectively optimal traits for domination of the marine benthos. Considering all metazoan taxa, the detection of 428 OCTUs on only two sites is likely a gross underestimate of actual metazoan richness. In all, 70% of Nematoda OCTUs were unique to Prestwick and 58–100% of the OCTUs for the other phyla were only present in Prestwick. In the absence of large-scale dispersal events sustaining ubiquitous meiobenthic communities [12] , levels of marine meiobenthic α-diversity, at the very least, in other parts of the world are likely to exceed expectations. Contrary to most morphological assessments of marine meiobenthic richness [34] , [35] , Platyhelminthes were consistently ranked as the second richest phylum in all the investigated samples. Platyhelminthes normally have to be identified from living or well-preserved material and their low ranking in other surveys perhaps arises from a global lack of taxonomic expertise, from extensive crypsis and from delicate body structures that do not survive harsh extraction methods. Given that the majority of free-living turbellarian Platyhelminthes encountered here occupy a top predacious role in benthic ecosystems [36] , the empirically demonstrated prominence of this phylum proves that conventional diversity assessments provide a notably distorted perspective of trophic relationships within the benthos [12] . Only six polychaete annelid OCTUs were identified, despite their dominance of benthic infaunal biomass [12] , [35] , probably because biomass dominance is affected by non-meiofaunal taxa (with only reproductive propagules and larvae being sampled here). Similarly, molluscan OCTUs comprised 21 bivalves and a single gastropod ( Littorina littorea ), likely representing larval and juvenile stages that are temporary members of the benthic meiofauna. Here, we also uncover a large percentage of OCTUs that have never been sequenced before, despite the nSSU region sampled here being the most frequently used genomic region for meiofaunal barcoding studies [37] , [38] . Some of our metagenetic sequences were clearly attributable to phylum, but were not closely related to previously sequenced taxa. Thus, we are likely to have uncovered a high level of phylogenetic novelty across a microgeographical scale that has not been shown from morphological or conventional DNA barcoding studies [15] of the meiobenthos. Quantifying biodiversity in species-rich environments raises questions of whether the sampling effort was sufficient to fully represent the natural community. Here, despite an extensive sampling strategy, the slope for OCTU rarefaction curves remained incomplete and the true standing diversity of an unremarkable Scottish beach is likely to exceed this estimate by an undetermined number of taxa. Such observations illustrate clearly the likely extent of marine meiofaunal diversity, and reveal that extensive sampling combined with ultrasequencing technologies makes realistic estimates of genetic diversity tractable in one of the largest ecosystems on earth. The present data offer novel insights into the organization, magnitude and identity of meiofaunal richness, but the mechanism of taxon delineation here warrants additional focus. In a multisite terrestrial survey, 60 times more traditional taxonomic scientific effort had to be expended in assigning only 10% of meiofaunal taxa to known species, compared with parallel studies that successfully assigned all vertebrate morphospecies to known taxa [39] . Lambshead [40] , using morphological taxonomy, spent 3 years describing 113 nematode morphospecies from the Firth of Clyde region (including the Prestwick sampling site), from approximately one-fifth of the volume of sediment analysed here. Our study identified 182 Nematoda OCTUs in approximately 3% of the time. Moreover, whereas the expertise of morphological taxonomists is, because of necessity, restricted to certain groups, high-throughput nSSU sequencing enables the simultaneous OCTU delineation of multiple phyla from large numbers of samples. Importantly, metagenetic analyses can also be linked retrospectively to morphospecies by using reverse taxonomy [41] . The approaches described provide a rapid, objective and cost-effective framework for exploring links between phyletic diversity, ecosystem structure and function. Such advances promise to substantially affect our ability to elucidate and predict the relationship between biodiversity and ecosystem function [42] , [43] , [44] : issues central to notions of resilience, recovery and sustainability [45] . Sample collection A total of 24 benthic samples were collected from the low-tide mark along an 800 m transect, using a standard corer methodology [46] , from marine sandy beach substrata in Prestwick (three every 100 m between 55°30.481′N, 4°37.489′W and 55°30.194′N, 4°37.368′W) and a further three from Littlehampton (50°48.021′N, 00°32.530′W), UK, during the summer of 2007. The latter sampling site was used as a geographically disparate out-group comparison. For the sequencing analysis, each biological sample comprised three pooled 44 mm diameter×100 mm benthic samples taken approximately 10 m apart. An additional core was taken for sediment analysis. All samples were immediately fixed in 500 ml storage pots containing 300 ml of DESS (20% DMSO and 0.25 M disodium EDTA, saturated with NaCl, pH 8.0) [47] . The meiofaunal size fraction was mechanically separated from the sand and concentrated by decanting five times with filtered tap water through a 45 μm filter. Subsequent separation from fine silt was achieved by repetitive centrifugation in 1.16 specific gravity LUDOX-TM solution [48] . Following centrifugation, each sample was retained on a distinct mesh sieve, which was then folded, sliced and placed in a 15 ml falcon tube and kept at −80 °C until DNA extraction. Samples were lysed overnight at 55 °C in lysis buffer (100 mM Tris–HCl, pH7.5; 100 mM NaCl; 100 mM EDTA; 1% SDS, 500 μg ml −1 proteinase K), assisted by spinning wheel mixing, and DNA extracted with the QIAamp DNA Blood Maxi Kit (Qiagen) following the manufacturer's protocol. Primer design and PCR strategy The genes coding for rRNA have been used for decades for the identification of microbial species [49] , [50] and are well suited for taxonomy, mainly because they are ubiquitous in cellular organisms, are of relatively large size, contain highly conserved and variable regions that facilitate primer design and are present in tandemly repeated, multiple copies enabling efficient PCR amplification [38] , [41] , [51] . For environmental metagenetic discovery, we chose the nSSU, as considerably more reference sequences are available in public databases for nSSU (1,246,462) than for the large subunit (LSU) (180,344) (ref. 52 ). Moreover, 'universal' nSSU primers have been shown to amplify more taxa from mock communities than from those designed for the LSU [17] . The 5′ region of the nSSU exhibits more segregating sites than the 3′ region in Metazoa [38] and so was selected as the target area for OCTU discrimination. MEGA version 4.1 (ref. 53 ) was used to align and compare a wide range of metazoan nSSU sequences with respect to existing degenerate primers and putative new priming sites spanning a region between 250 and 500 bp in length (a combination of average mean read length and maximum permitted amplicon size of a 454 Life Sciences, Roche Applied Science GSFLX amplicon sequencing run). Of all primer permutations, SSU_FO4 (5′-GCTTGTCTCAAAGATTAAGCC-3′) and SSU_R22 (5′-GCCTGCTGCCTTCCTTGGA-3′) [14] primers were selected, as they exhibited pronounced homology across meiofaunal phyla, but also flanked a highly divergent region of the nSSU and were used for subsequent amplicon generation. Fusion primers were then developed in which a proprietary primer sequence (Adaptor A or B) of the Roche 454 GSFLX sequencing technology and a sample-specific five nucleotide key tag (to differentiate between multiple samples) were included [54] . All fusion primers were designed using PRIMER PREMIER 5.0 (Premier Biosoft International), considering physical and structural properties of the oligonucleotides (such as annealing temperature, G+C percentage, hairpins and false priming). The forward fusion primers were ∼ 45 bases in length and designed such that the 454 A-adaptor is followed by the tag (each of which differed by at least two bases) [54] , and then by the experimental forward primer (SSU_FO4). The reverse primers were designed similarly, to optimize thermal compatibility. PCR amplification of the specified nSSU region was performed using 1 μl of genomic DNA template (1:500 dilutions) in 3 × 40 μl reactions using Pfu DNA polymerase (Promega). PCR conditions involved a 2 min denaturation at 95 °C followed by 35 cycles of 1 min at 95 °C, 45 s at 57 °C, 3 min at 72 °C and a final extension of 10 min at 72 °C. Negative controls (ultrapure water only) were included for all amplification reactions. Electrophoresis of triplicate PCR products was undertaken on a 2% gel with Top Vision LM GQ Agarose (Fermentas), and the expected 450 bp fragment was purified using the QIAquick Gel Extraction Kit (Qiagen), following the manufacturer's instructions, before pooling identical samples. All purified PCR products were then quantified with an Agilent Bioanalyser 2100, diluted to the same concentration, pooled together to create a single sample and sequenced in one direction (A-Amplicon) on half a plate of a Roche 454 GSFLX (454 Life Sciences, Roche Applied Science) sequencing platform at Liverpool University's Centre for Genomic Research, UK. Further details regarding the rationale, theory and execution of environmental metagenetic analyses of the meiofaunal biosphere can be found in Creer et al . [7] Sediment analysis Particle size analysis was carried out using a Malvern Mastersizer 2000, which uses laser diffraction to calculate the particle size distribution for individual sediment grains in the range 0.02–2,000 μm. To prevent flocculation, before testing, the samples were immersed for 24 h in distilled water with added dispersant (sodium hexametaphosphate). The Mastersizer determines particle size distribution by volume and the results of the particle size analysis are reported as the cumulative median grain size. Data analysis Sequences generated from the Roche 454 GSFLX pyrosequencing were analysed using the OCTUPUS pipeline (supplementary software available at http://octupus.sourceforge.net/ ). Briefly, OCTUPUS comprises a number of Perl scripts that concatenate quality trimming [55] , tag matching and size culling, before the assignation of user-defined substitutional difference-based cutoff clustering. The clustering module of OCTUPUS involves three steps. Initially, sequences are compared successively with each other by MEGABLAST [56] to define different OCTU groups, separated by a user-defined genetic distance. If an unassigned sequence matches an existing OCTU sequence (for example, 97% similarity or more), the companion sequences are aligned using MUSCLE [23] , and if the resulting consensus sequence differs from the original alignment, the consensus OCTU sequence is changed to reflect the diversity of sequences within the OCTU cluster. If the consensus OCTU does not change following a preset number of novel comparisons, further consensus OCTU matching sequences will be placed within the OCTU cluster, bypassing a computationally intractable number of multiple sequence alignments that would otherwise be required in the analysis of large metagenetic data sets. Benchmarking trials have shown that 10 additions to the OCTU cluster without consensus amendment provide a stable estimate of OCTU numbers and were used throughout in this study. OCTUs were annotated using MEGABLAST (megablast -d database path -D 2 -p 90 -a 2 -b 1 -v 1 -i infile -F F>outfile) against the downloaded GenBank/EMBL/DDBJ nucleotide database and taxonomic annotation was restricted to matches of 90% and higher. Acknowledging concerns regarding the misinterpretation of levels of richness due to the formation of recombinant DNA molecules in environmental DNA sequencing [26] , [57] , we adopted an aggressive putative chimera culling regime embedded within the OCTUPUS pipeline for the primary data set [7] . The OCTUPUS chimera screening was followed by manual removal of putative false positive OCTUs (that is, those that exhibited more than 10 base pair mismatches with the MEGABLAST reference sequence) and retrieval of clear false-negative chimeras (that is, those that exhibited 100% length matches with already sequenced taxa). To compare independent estimates of taxon richness, the OCTUPUS clustering algorithm was also tested against the HCluster algorithm of ESPRIT [13] on a subsample of the larger data set. Finally, OCTU richness generated from the above OCTUPUS algorithm was benchmarked at a range of percentage similarity cutoff against a reference data set comprising the metagenetic analysis of a phylogenetically diverse combination of 41 nematode [17] species. Scripts for preprocessing the above data are available from the Natural Environment Research Council's Environmental Bioinformatics Centre Script Repository ( http://nebc.nerc.ac.uk/tools/scripts/general-bioinformatics ). For the 54 OCTUs exhibiting BLAST hits below 90% identity, manual MEGABLAST searches were conducted and phylogenetic affinities investigated by means of the NCBI taxonomy browser. Sequence data and all associated fusion primer codes have been deposited in the Entrez short read archive under accession number SRA009394. For direct ecological comparisons of between-sample OCTU richness, the original data set was reanalysed using 15,000 randomly picked sequences (over 200 bases in length, n =135,000) from each sample, before OCTUPUS clustering and annotation. The total number of OCTUs generated from the original and standardized data sets was significantly correlated (Spearman's coefficient: ρ =0.783, P =0.0132); nevertheless, interpretations derived from direct comparisons of richness between samples refer to the standardized data set. Sample cluster analyses (UPGMA) were performed using the Multivariate Statistical Package [58] using Sorensen's Coefficient on a binary (presence/absence of OCTU) data matrix. Phylum-specific rarefaction curves for the Prestwick transect were generated using EstimateS (Version 8.2.0, R.K. Colwell) using a range of estimators (for example, ACE, Chao1, Jackknife1 and Bootstrap) that yielded very similar results. The ACE abundance-based coverage estimator [59] was used because it represents a consensus view of the analyses and has proven to work well for the analysis of metagenetic data sets [3] . Accession number: All sequences and associated fusion primer codes have been deposited in the Entrez short read archive under accession number SRA009394. How to cite this article: Fonseca, V.G. et al . Second-generation environmental sequencing unmasks marine metazoan biodiversity. Nat. Commun. 1:98 doi: 10.1038/ncomms1095 (2010).